Phosphoinositide 3-kinase p110δ promotes lumen formation through the enhancement of apico-basal polarity and basal membrane organization Signalling triggered by adhesion to the extracellular matrix plays a key role in the spatial orientation of epithelial polarity and formation of lumens in glandular tissues. Phosphoinositide 3-kinase signalling in particular is known to influence the polarization process during epithelial cell morphogenesis. Here, using Madin–Darby canine kidney epithelial cells grown in 3D culture, we show that the p110δ isoform of phosphoinositide 3-kinase co-localizes with focal adhesion proteins at the basal surface of polarized cells. Pharmacological, siRNA- or kinase-dead-mediated inhibition of p110δ impair the early stages of lumen formation, resulting in inverted polarized cysts, with no laminin or type IV collagen assembly at cell/extracellular matrix contacts. p110δ also regulates the organization of focal adhesions and membrane localization of dystroglycan. Thus, we uncover a previously unrecognized role for p110δ in epithelial cells in the orientation of the apico-basal axis and lumen formation. Apical-basal polarity is a fundamental feature of epithelial cells required for the structural and functional integrity of the epithelial tissue [1] , [2] . Conversely, the disruption of polarity in epithelial cells is often associated with infectious diseases and cancer [3] . Apical-basal polarity is initiated by signalling from cell–cell and cell-to-extracellular matrix (ECM) contacts [4] , [5] . Events such as intracellular trafficking [6] , cytoskeletal organization [7] and actions of evolutionary conserved complexes mediate further development of the apical and basolateral membrane domains [8] . Several recent reports have demonstrated that mechanical factors are also important regulators of cell polarity [9] , [10] . Establishment of polarity in epithelial cells results in the segregation of plasma membrane in an apical domain facing the outside surface of the body, or the lumen of internal cavities, and the basolateral domain oriented away from the lumen [11] . The phosphoinositide 3-kinase (PI3K) family of lipid kinases is divided into three different classes based on primary structure, regulation and lipid substrate specificity. The class I PI3Ks are the best characterized and are frequently deregulated in cancer [12] . Mammals have four Class I PI3K isoforms, all of which are heterodimeric PI3K enzymes consisting of a regulatory subunit in complex with a 110-kDa catalytic subunit, either p110α (PI3Kα), β (PI3Kβ), γ (PI3Kγ) or δ (PI3Kδ). p110α and p110β are ubiquitously expressed, whereas p110γ and p110δ are enriched in cells of haematopoietic lineage [13] . All class I PI3Ks produce the phosphatidylinositol(3,4,5)-triphosphate (PtdIns(3,4,5)P 3 ) lipid that controls a complex cellular signalling network, with crucial roles in regulation of apico-basal polarity and epithelial cell morphogenesis [14] , [15] , [16] , [17] , [18] . PtdIns(3,4,5)P 3 signals can be terminated through the action of the 3-phosphatase PTEN or the 5-phosphatases SHIP1/2 to produce PtdIns(4,5)P 2 and PtdIns(3,4)P 2 , respectively [19] , [20] . In polarized epithelial cells, PtdIns(3,4,5)P 3 and PI3Ks are mainly present on the basolateral membrane [21] , while PTEN plays a central role in the formation of the apical membrane [22] . We have recently reported that SHIP2 is present at the basolateral membrane and regulates cell polarization [23] . Although the involvement of PtdIns(3,4,5)P 3 has previously been established in the polarization of epithelial cells, the underlying mechanisms and the function of the specific PI3K isoforms in this process have not yet been addressed. Here we demonstrate the presence of p110δ at the basolateral membrane of polarized MDCK cysts. Our data also reveal that p110δ is required to orient the apical-basal axis and lumen formation through both focal adhesions and basal membrane organization. p110δ activity controls apico-basal axis and lumen formation All class I PI3K isoforms generate PtdIns(3,4,5)P 3 and thus the kinase activity of individual PI3K isoforms cannot be readily distinguished in cells by detection of their lipid product or by using broad-spectrum PI3K inhibitors such as wortmannin and LY294002. We therefore tested ATP-competitive isoform-selective inhibitors of PI3K (ref. 24 ) on apico-basal polarity of MDCK grown in three-dimensional (3D) as a model system. These include PI-103, a multi-targeted inhibitor for p110α/β/δ/γ, which inhibits p110α most efficiently but also targets p110β at 10 to 30-fold higher concentrations, and the isoform-selective inhibitors AS-605240, TGX115 and IC87114 that target p110γ, p110β/p110δ and p110δ, respectively. The specificity profile of these compounds was previously determined by measuring IC 50 values in vitro against purified PI3K family members [24] . We also used CAL-101, now called Idelalisib, a derivative of IC87114 with increased potency, which is in clinical trials for B-cell malignancies [25] , [26] . To test these pharmacological inhibitors on apico-basal polarity, single MDCK cells were grown on matrigel to form cysts. Twenty-four hours after plating, cells were treated or not with the different PI3K inhibitors for 72 h, followed by confocal microscopy analysis. In non-treated control cysts, β-catenin staining revealed a monolayer of polarized cells surrounding an open central lumen as visualized by the apical marker podocalyxin (PCX; Fig. 1a , left panel). Following the localization of PCX enabled the investigation of the impact of PI3K inhibition on the establishment of epithelial apico-basal polarity. The four major phenotypes (multi-lumens, no lumen, small and inverted polarized cysts) obtained following treatments with the different inhibitors are represented in Fig. 1a . The percentages of each phenotype depending on the concentrations of inhibitors were gathered in the Supplementary Fig. 1 and presented as pie charts in Fig. 1b . Cysts treated with PI-103 showed a dose-dependent change in lumen formation and cyst growth. At a concentration of 10 μM, 62.33% of the cysts presented no lumen and were very small in size. AS-605240, a selective p110γ inhibitor, had effects similar as PI-103 even though the number of small cysts was reduced (36.68% at 10 μM). Treatment of cysts with TGX115 led to the formation of cysts with multi-lumens and no lumen. Moreover, a small proportion (6.52% at 10 μM) of cysts with inverted polarity was seen, detected via the persistence of PCX localized at the cyst periphery. Treatment with the p110δ inhibitor IC87114 increased the number of cysts with inverted polarity significantly in a dose-dependent manner, from 3.14 to 34.31% at 0.1 μM and 10 μM of IC87114, respectively. These data were confirmed using CAL-101 (Idelalisib), another specific inhibitor of the p110δ. Together these data indicated that all the isoforms of class I PI3K participate in the establishment of epithelial cell polarity. However, only the inhibition of p110δ elicited an inversion of apico-basal polarity in a population of cysts, which is suggestive of a specific role of the latter isoform of PI3K in the establishment of the apico-basal polarity axis. 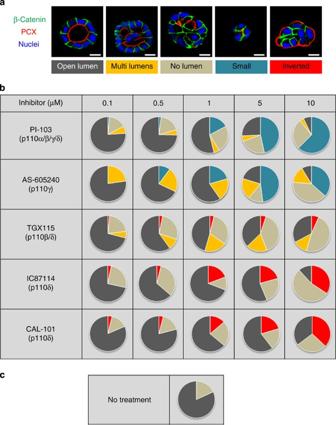Figure 1: p110δ activity is required for polarity in MDCK cysts. (a) MDCK cells, plated on Matrigel to form cysts, were treated 24 h after plating with different p110 inhibitors: PI-103 (inhibitor of p110α, β, γ and δ), AS-605240 (inhibitor of p110γ), TGX115 (inhibitor of p110β and δ), IC87114 and CAL-101 (inhibitors of p110δ). Inhibitors were used at different concentrations (0–10 μM). Cysts were grown for another 72 h with a daily change of the medium containing inhibitor. Cysts presented different phenotypes (Normal lumen, multi-lumen, no lumen, small cysts with no lumen and inverted polarity). These phenotypes were identified by staining β-catenin in green, PCX in red and Hoechst (blue) as indicated in the pictures. A confocal section through the middle of cyst is shown. Scale bar, 10 μm. (b) The table shows a schematic representation of phenotype at different concentrations. Colour for each phenotype in pie is corresponding to the color below pictures ina. (c) The same representation as inbfor cells not treated. Figure 1: p110δ activity is required for polarity in MDCK cysts. ( a ) MDCK cells, plated on Matrigel to form cysts, were treated 24 h after plating with different p110 inhibitors: PI-103 (inhibitor of p110α, β, γ and δ), AS-605240 (inhibitor of p110γ), TGX115 (inhibitor of p110β and δ), IC87114 and CAL-101 (inhibitors of p110δ). Inhibitors were used at different concentrations (0–10 μM). Cysts were grown for another 72 h with a daily change of the medium containing inhibitor. Cysts presented different phenotypes (Normal lumen, multi-lumen, no lumen, small cysts with no lumen and inverted polarity). These phenotypes were identified by staining β-catenin in green, PCX in red and Hoechst (blue) as indicated in the pictures. A confocal section through the middle of cyst is shown. Scale bar, 10 μm. ( b ) The table shows a schematic representation of phenotype at different concentrations. Colour for each phenotype in pie is corresponding to the color below pictures in a . ( c ) The same representation as in b for cells not treated. Full size image To validate this proposition, we further investigated the effect of IC87114 at 10 μM on the different stages of lumen formation ( Fig. 2a ) as described in a previous report [27] . As presented in the top panels of Fig. 2a when plating individual MDCK cells in 3D culture at the early stage of cyst formation, PCX initially localized at the ECM-contacting surface in early aggregates with β-catenin accumulating at cell–cell junctions. As cysts develop polarity, PCX is displaced at the centre of the cell–cell contact at a site called the apical membrane initiation site (AMIS). The lumen then starts to develop at a site termed the ‘pre-apical patch’ (PAP) at 48 h of culture and becomes visible at 72 h and then continues to develop as seen at 96 h of culture ( Fig. 2a ). In striking contrast to control cysts, on treatment with IC87114, PCX was found to remain at the ECM surface until 96 h, while the cells continued to proliferate and maintain cell-to-cell contacts as shown by β-catenin and nuclei staining ( Fig. 2a ). We also analysed the localization of the tight junction protein Zonula occludens protein 1 (ZO-1) at the early stages of lumen formation. As observed for PCX, treatment with IC87114 resulted in the inappropriate accumulation of ZO-1 at the cell periphery, while tight junctions formed at the apico-lateral boundary in control cysts ( Fig. 2b ). Statistical analysis of the impact of p110δ inhibition on the observed lumen morphologies indicated a significant decrease in the proportion of cysts with a central lumen (or lumen precursor) regardless of days in culture ( Fig. 2c ). These data strongly suggest that the enzymatic activity of p110δ is required to orient the apico-basal polarity axis and to drive the formation of AMIS, which is necessary for lumen formation. 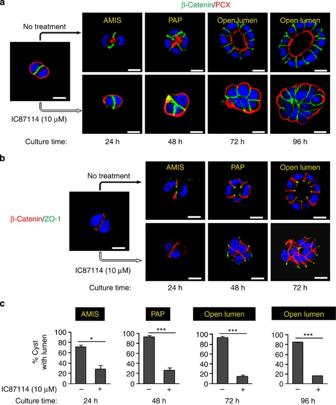Figure 2: p110δ activity is required for lumen initiation in MDCK cysts. (a) Time course analysis of polarity and lumen formation in MDCK cells, treated or not with 10 μM of IC87114 and plated on Matrigel to form cysts, fixed and stained after 24, 48, 72 and 96 h of culture, corresponding to different stages of lumen formation: PAP, pre-apical patch and open lumen. Cells were stained for β-catenin (green) and PCX (red) and a single confocal section through the middle of cyst is shown. Scale bar, 10 μm. (b) Cells were grown as inaand analysed after 24, 48 and 72 h of culture and stained for β-catenin (red) and ZO-1 (green) and a single confocal section through the middle of cyst is shown. Scale bar, 10 μm. (c) Percentage of MDCK cysts with AMIS, PAP or open lumen from three independent experiments were presented in histograms. Values are expressed as mean±s.e.m. *P<0.05, ***P<0.0001 (Student’st-test). Figure 2: p110δ activity is required for lumen initiation in MDCK cysts. ( a ) Time course analysis of polarity and lumen formation in MDCK cells, treated or not with 10 μM of IC87114 and plated on Matrigel to form cysts, fixed and stained after 24, 48, 72 and 96 h of culture, corresponding to different stages of lumen formation: PAP, pre-apical patch and open lumen. Cells were stained for β-catenin (green) and PCX (red) and a single confocal section through the middle of cyst is shown. Scale bar, 10 μm. ( b ) Cells were grown as in a and analysed after 24, 48 and 72 h of culture and stained for β-catenin (red) and ZO-1 (green) and a single confocal section through the middle of cyst is shown. Scale bar, 10 μm. ( c ) Percentage of MDCK cysts with AMIS, PAP or open lumen from three independent experiments were presented in histograms. Values are expressed as mean±s.e.m. * P <0.05, *** P <0.0001 (Student’s t -test). Full size image p110δ is expressed at the basolateral membrane The results described above indicated a crucial function of p110δ in establishment of cell polarity. p110δ is known to be mainly expressed in cells of the haematopoietic lineage, and although several studies have reported expression in epithelial cells [28] , [29] , its possible role in epithelial morphogenesis has not been determined. Thus, we decided to further characterize the p110δ protein expression and localization in MDCK cells. First, we examined by immunoblot the expression of p110δ in MDCK cells using as a positive control a lysate from HeLa cells, a non-leukocyte cell that is known to express high levels of p110δ (refs 13 , 30 ). A 110-kDa protein was detected in both cell lines; however, the intensity of the signal was very weak in MDCK cells ( Supplementary Fig. 2a ; the specific band is marked with an arrow), which is in line with the quantitative reverse transcription–PCR (qRT–PCR) analysis for p110δ mRNA abundance in these cells ( Supplementary Fig. 2b ). The amplified qRT–PCR product from MDCK cells presented a product of the same size as the product isolated from HeLa cells ( Supplementary Fig. 2c ) and with similarity to the p110δ canine sequence, as shown in ( Supplementary Fig. 2d ). Then we examined the presence of the different class I PI3K isoforms in MDCK cells using qRT–PCR. Data presented in Supplementary Fig. 2e indicated that the p110β isoform was the most highly expressed. Together these results indicated the presence of the p110δ in MDCK cells. Next we validated the antibody and the subcellular localization of p110δ in polarized MDCK cells through transfection of the cells with different p110δ constructs. First, MDCK cells were transfected using an untagged p110δ cDNA (UT-p110δ) and the efficiency of the transfection was validated by immunoblot analysis ( Fig. 3a ) using a p110δ-specific antibody (sc: anti-p110δ). In transfected cells, we observed an intense signal at 110 kDa corresponding to the size of the signal observed in the lysate of HeLa cells, used here as a positive control. In parallel, we assessed the subcellular localization of the exogenous p110δ protein in transfected cells plated to form cysts in matrigel culture ( Fig. 3b ). Staining of the aforementioned cysts with one of the commercially available p110δ-specific antibodies (sc: Anti-p110δ) revealed a basolateral signal in both control and the untagged p110δ cDNA transfected cells, as expected. As anticipated, based on the results of the immunoblotting analysis using this antibody ( Fig. 3a ), the signal was weaker in control cells when compared with the transfected cells ( Supplementary Fig. 3 ). Similar results were obtained using a different commercial antibody raised against p110δ (ab: anti-p110 δ; Supplementary Fig. 3 ; Fig. 3b ). On the basis of these immunolocalization data, it was determined that the antibody from Abcam was more appropriate for downstream immunofluoresence studies because of the higher signal intensity achieved using this reagent in these cells. Next we used Myc-tagged p110δ cDNAs expressed from two different expression vectors (Myc1-p110δ, Myc2-p110δ, see methods). Immunoblot analysis revealed that the two exogenous proteins were detected with both p110δ- and Myc-specific antibodies as shown in Fig. 3c and Supplementary Fig. 4a , respectively, for Myc2-p110δ and Myc1-p110δ. Furthermore, we used the Myc tag and p110δ antibodies to analyze by immunofluorescence the cysts from cells transfected or not (Ctrl) with Myc2-p110δ cDNA. The two antibodies specifically labelled the Myc-tagged-p110δ protein at the basolateral membrane ( Fig. 3d ). The signal of p110δ expression in the Myc2-p110δ expressing cysts was measured by ImageJ analysis and compared to endogenous p110δ signal ( Fig. 3e ). These data confirmed a significantly increased signal intensity of p110δ on enforced expression of exogenous protein ( Fig. 3e ). 3D reconstructions for Ctrl and Myc2-p110δ cysts were presented in Fig. 3d . Basolateral localization was also observed for Myc1-tagged p110δ ( Supplementary Fig. 4b ). Thus, together these data indicated that p110δ-specific antibodies detected both endogenous and the exogenous proteins. We concluded that the localization of exogenous p110δ is similar to the subcellular distribution observed for the endogenous protein at the basolateral membrane. Co-staining of p110δ in Myc2-p110δ-expressing cysts with β-catenin indicated that the distribution pattern of p110δ is different from that of β-catenin, which is mainly present in the lateral domain ( Supplementary Fig. 4c ). 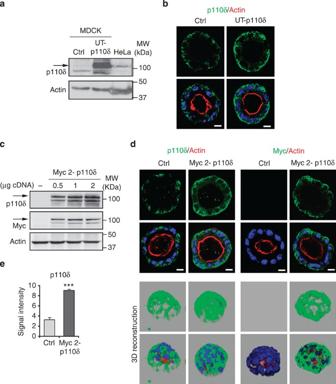Figure 3: p110δ localization at the basolateral membrane of MDCK cysts. (a) Immunoblot analysis of p110δ in MDCK transfected or not with 1 μg of untagged p110δ cDNAs (UT-p110δ), using p110δ-specific antibody (sc7176). HeLa cells are positive control for p110δ and actin was used as a loading control. (b) MDCK cells inawere grown in Matrigel to form cysts and then stained for p110δ (green) using p110δ-specific antibody (ab32401), actin (red) and Hoechst (blue) as indicated in the pictures. Single confocal section through the middle of cyst is shown. Scale bar, 10 μm. (c) Immunoblot analysis of MDCK transfected or not with different amounts (0.5, 1 and 2 μg) of Myc-tagged-p110δ cDNA (Myc 2-p110δ) and revealed with p110δ (sc7176) and myc tag antibodies. Actin was used as a loading control. (d) Cells incwere grown in Matrigel to form cysts and then stained for p110δ using p110δ-specific antibody (ab32401) or Myc (green), actin (red) and Hoechst (blue) as indicated in the pictures. Single confocal section through the middle of a cyst is shown. Scale bar, 10 μm. A 3D reconstruction from allxzsections is presented in the bottom panel. (e) Quantification of p110δ intensity by ImageJ from 20 cysts from three independent experiments, values are expressed as mean±s.e.m., ***P<0.0001 (Student’st-test). Figure 3: p110δ localization at the basolateral membrane of MDCK cysts. ( a ) Immunoblot analysis of p110δ in MDCK transfected or not with 1 μg of untagged p110δ cDNAs (UT-p110δ), using p110δ-specific antibody (sc7176). HeLa cells are positive control for p110δ and actin was used as a loading control. ( b ) MDCK cells in a were grown in Matrigel to form cysts and then stained for p110δ (green) using p110δ-specific antibody (ab32401), actin (red) and Hoechst (blue) as indicated in the pictures. Single confocal section through the middle of cyst is shown. Scale bar, 10 μm. ( c ) Immunoblot analysis of MDCK transfected or not with different amounts (0.5, 1 and 2 μg) of Myc-tagged-p110δ cDNA (Myc 2-p110δ) and revealed with p110δ (sc7176) and myc tag antibodies. Actin was used as a loading control. ( d ) Cells in c were grown in Matrigel to form cysts and then stained for p110δ using p110δ-specific antibody (ab32401) or Myc (green), actin (red) and Hoechst (blue) as indicated in the pictures. Single confocal section through the middle of a cyst is shown. Scale bar, 10 μm. A 3D reconstruction from all xz sections is presented in the bottom panel. ( e ) Quantification of p110δ intensity by ImageJ from 20 cysts from three independent experiments, values are expressed as mean±s.e.m., *** P <0.0001 (Student’s t -test). Full size image p110δ membrane localization depends on its enzymatic activity In subsequent experiments, we analysed p110δ protein cellular localization during cystogenesis ( Fig. 4 ) and we confirmed its basolateral staining at the different stages of cyst formation ( Fig. 4a ). Treatment with IC87114 induced the displacement of p110δ from the membrane at the ECM contact site to the cytoplasm as demonstrated by analysis of the p110δ staining signal using imageJ (see Methods; Fig. 4b,c ). We next sough to evaluate the effect of IC87114 on the exogenous Myc-tagged-p110δ membrane localization ( Fig. 4d ). Similar to the endogenous protein, IC87114 treatment significantly decreased the membrane signal of Myc with a concomitant shift into the cytoplasmic area ( Fig. 4e ). 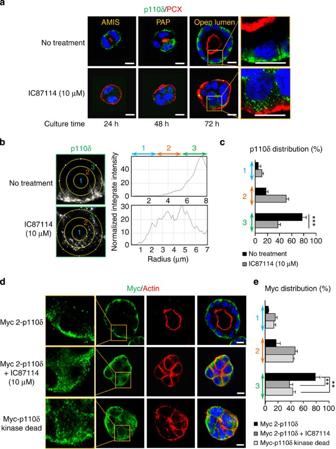Figure 4: p110δ localization at the basolateral membrane of MDCK cysts depends on its activity. (a) Time course analysis of p110δ in MDCK cells grown on Matrigel to form cysts and treated or not with IC87114 at 10 μM. Cysts were fixed and stained after 24, 48 and 72 h of culture. Immunostaining was performed for p110δ (green) using p110δ-specific antibody (ab32401), PCX (red) and Hoechst (blue) as indicated on the pictures. Single confocal section through the middle of cyst is shown. Scale bar, 10 μm. A higher magnification of the data from 72 h of culture is presented in the right column. (b) The distribution of p110δ signal was analysed by ImageJ software in an individual cell from a cyst. A circle was defined at the periphery of each cell and the plugin produces a profile plot of normalized integrated intensities around concentric circles as a function of distance from a point in the image, considered here as the centre of the cell. The circle was divided in three bands (1, 2, 3) with equal radius. (c) The total intensity in each band was calculated from 20 cells and is represented as a histogram. values are expressed as mean±s.e.m. ***P<0.0001 (Student’st-test). (d) MDCK cells transfected with 1 μg of Myc 2-p110δ cDNA were treated or not with 10 μM of IC87114. MDCK cells were also transfected with 1 μg of Myc-p110 kinase-dead (KD) cDNA. Immunostaining was performed for Myc (green), actin (red) and Hoechst (blue) as indicated on the pictures. Single confocal section through the middle of the cyst is shown. A higher magnification of the data is presented in the right column. Scale bar, 10 μm. (e) The distribution of Myc signal was analysed by ImageJ software in an individual cell from a cyst as inb, and total intensity in each band calculated from 20 cells was represented as histogram. values are expressed as mean±s.e.m. **P<0.001 (Student’st-test). Figure 4: p110δ localization at the basolateral membrane of MDCK cysts depends on its activity. ( a ) Time course analysis of p110δ in MDCK cells grown on Matrigel to form cysts and treated or not with IC87114 at 10 μM. Cysts were fixed and stained after 24, 48 and 72 h of culture. Immunostaining was performed for p110δ (green) using p110δ-specific antibody (ab32401), PCX (red) and Hoechst (blue) as indicated on the pictures. Single confocal section through the middle of cyst is shown. Scale bar, 10 μm. A higher magnification of the data from 72 h of culture is presented in the right column. ( b ) The distribution of p110δ signal was analysed by ImageJ software in an individual cell from a cyst. A circle was defined at the periphery of each cell and the plugin produces a profile plot of normalized integrated intensities around concentric circles as a function of distance from a point in the image, considered here as the centre of the cell. The circle was divided in three bands (1, 2, 3) with equal radius. ( c ) The total intensity in each band was calculated from 20 cells and is represented as a histogram. values are expressed as mean±s.e.m. *** P <0.0001 (Student’s t -test). ( d ) MDCK cells transfected with 1 μg of Myc 2-p110δ cDNA were treated or not with 10 μM of IC87114. MDCK cells were also transfected with 1 μg of Myc-p110 kinase-dead (KD) cDNA. Immunostaining was performed for Myc (green), actin (red) and Hoechst (blue) as indicated on the pictures. Single confocal section through the middle of the cyst is shown. A higher magnification of the data is presented in the right column. Scale bar, 10 μm. ( e ) The distribution of Myc signal was analysed by ImageJ software in an individual cell from a cyst as in b , and total intensity in each band calculated from 20 cells was represented as histogram. values are expressed as mean±s.e.m. ** P <0.001 (Student’s t -test). Full size image Finally, we used the kinase-dead mutant (R894P) of p110δ (Myc-p110δ kinase-dead) to validate the effects of the pharmacological inhibitors. MDCK cells were transfected with the corresponding cDNA and grown on matrigel to form cysts. Myc-p110δ kinase-dead protein, revealed with Myc antibody, was significantly localized in the cytoplasm ( Fig. 4d,e ) demonstrating that membrane localization of p110δ is dependent on its enzymatic activity. Of interest, these cells expressing the mutant protein formed inverted polarized cyst (about 29%) with actin present at the cell periphery, while in control cysts actin marks the central lumen ( Fig. 4d ). These data are analogous to those obtained with treatment of cells using CAL-101 or IC87114 ( Fig. 1 ) and confirmed the requirement of active p110δ to orient polarity and allow lumen formation. PtdIns(3,4,5)P 3 , monitored using a specific antibody, was mainly observed at the basolateral membrane, in line with previous studies using the PH domain of Akt as a PtdIns(3,4,5)P 3 probe [21] . In accordance with the observations made for the p110δ protein localization in cysts ( Supplementary Fig. 4d,e ), inhibition of its activity significantly reduced the observed PtdIns(3,4,5)P 3 membrane localization with a concomitant shift of the immunoreactive population to a cytoplasmic pool. Taken together, these results strongly suggest that localization of the majority of PtdIns(3,4,5)P 3 at the basal membrane in MDCK cysts is dependent on p110δ kinase activity. p110δ controls Rac1 activation and BM assembly Cell contacts with the ECM trigger numerous signalling events that provide the initial cue to define the polarity axis. The laminins are major and important biologically active components of the basement membrane (BM), a thin layer of ECM underlying the epithelial cells. Several publications have now reported the crucial role of laminins in orientation of apico-basal polarity axis through the activation of Rac1 (refs 31 , 32 , 33 , 34 ). PI3Ks are important regulators of Rac1 (refs 21 , 35 ) and its implication in Rac1-mediated regulation of lumen formation has been evoked [36] . Therefore, and according to the observed effects of p110δ inhibition on orientation of the apico-basal axis, we evaluated Rac1 activation and, importantly, it is increased with lumen formation. Rac1 activation was significantly reduced by treatment of cysts with IC87114 ( Supplementary Fig. 5 ), suggesting that p110δ activity could affect activation of Rac1. Next we examined the possible role of p110δ activity on laminin assembly. As presented in Fig. 5a , (the xz section was presented below each picture and the 3D reconstruction was shown on the right part of the panel), laminin was visible at the cyst periphery and formed a prominent structure covering the control cysts that disappeared on treatment of cells with IC87114, while laminin was still present in the culture gel. Under such conditions, PCX is externalized (red staining) and further confirms the inverted polarization of the IC87114 treated cysts. The treatment of cysts with CAL-101 led to data similar to those obtained using IC87114. Then, we analysed laminin staining in cysts from MDCK cells expressing the Myc-p110δ kinase-dead mutant ( Fig. 5b ) and no laminin was found surrounding these cysts suggesting that the recruitment of laminin at the site of cell contact with the ECM required p110δ activity. Along with laminins, type IV Collagen is a key ECM protein, essential for maintaining the structural integrity of BM [37] . Accordingly, we also analysed type IV Collagen assembly in the system. Of interest, the treatment of cysts with IC87114 or CAL-101 removed the layer of type IV Collagen underlying the cysts as observed in controls ( Fig. 5c ). Taken together, these results strongly suggested that p110δ is necessary for the assembly of the BM at the cell surface and that it probably fulfills this role by regulation of a signalling pathway that involved Rac 1 activation. 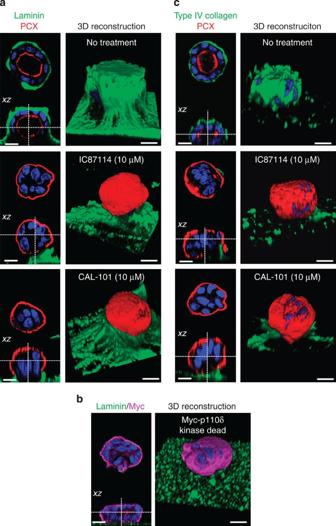Figure 5: Laminin and type IV collagen assembly is dependent on p110δ activity. (a) MDCK cells treated or not with 10 μM of p110δ inhibitors (IC87114 or CAL-101) were grown on matrigel for 4 days to form cysts and then fixed and stained with laminin (green), PCX (red) and Hoechst (blue) as indicated on the pictures. A confocal section through the middle of the cyst is shown and thexzsection is presented below each panel. Scale bar, 10 μm. 3D reconstruction from allxzsections is presented in the right column. (b) MDCK cells transfected or not with 1 μg of Myc-p110δ KD were grown on matrigel for 4 days to form cysts and then fixed and stained with laminin (green), Myc (purple) and Hoechst (blue) as indicated on the pictures. A confocal section through the middle of cyst is shown andxzsection is presented below each panel. Scale bar, 10 μm. 3D reconstruction from allxzsections is presented in the right column. (c) Cells treated as inastained with type IV collagen (green), PCX (red) and Hoechst (blue) as indicated in the pictures. A confocal section through the middle of the cyst is shown and thexzsection is presented below each panel. Scale bar, 10 μm. 3D reconstruction from allxzsections is presented in the right column. Figure 5: Laminin and type IV collagen assembly is dependent on p110δ activity. ( a ) MDCK cells treated or not with 10 μM of p110δ inhibitors (IC87114 or CAL-101) were grown on matrigel for 4 days to form cysts and then fixed and stained with laminin (green), PCX (red) and Hoechst (blue) as indicated on the pictures. A confocal section through the middle of the cyst is shown and the xz section is presented below each panel. Scale bar, 10 μm. 3D reconstruction from all xz sections is presented in the right column. ( b ) MDCK cells transfected or not with 1 μg of Myc-p110δ KD were grown on matrigel for 4 days to form cysts and then fixed and stained with laminin (green), Myc (purple) and Hoechst (blue) as indicated on the pictures. A confocal section through the middle of cyst is shown and xz section is presented below each panel. Scale bar, 10 μm. 3D reconstruction from all xz sections is presented in the right column. ( c ) Cells treated as in a stained with type IV collagen (green), PCX (red) and Hoechst (blue) as indicated in the pictures. A confocal section through the middle of the cyst is shown and the xz section is presented below each panel. Scale bar, 10 μm. 3D reconstruction from all xz sections is presented in the right column. Full size image ECM regulates p110δ expression To further characterize the interplay between PI3K and ECM, first MDCK cells were transfected with Myc-tagged p110δ cDNA (Myc2-p110δ) and plated on matrigel to form cysts, then laminin and type IV Collagen distributions were assessed at the different stages of cystogenesis. As presented in Fig. 6a , laminin was visible at the cyst periphery and the signal significantly increased from the AMIS stage (24 h of culture) to large lumen at 96 h of culture ( Fig. 6a,b ). The laminin layer surrounding the cysts became thicker whatever the stage of polarization was due to the enforced expression of Myc 2-p110δ ( Fig. 6a,b ). These data are consistent with those obtained from the analysis type IV Collagen distribution in these cysts ( Fig. 6c,d ). 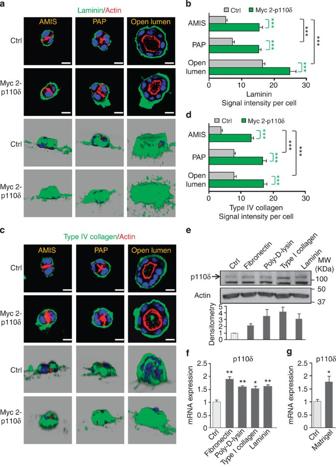Figure 6: ECM regulates p110δ expression. (a) MDCK cells transfected or not with 1 μg of Myc 2-p110δ were grown on matrigel and fixed after 24 h for AMIS, after 48 h for PAP and after 72 h for open lumen. Cells were stained with laminin (green), actin (red) and Hoechst (blue) as indicated in the pictures. A confocal section through the middle of cyst is shown. Scale bar, 10 μm. 3D reconstruction from allxzsections is presented in a grey background. Laminin signal intensity of individual cell is analysed with ImageJ software for 30 cells and represented as histogram inb. Values are expressed as mean±s.e.m. ***P<0.0001 (Student’st-test). (c,d) Same asaandb, respectively, for type IV collagen staining (green) and signal intensity. (e) MDCK cells grown for 24 h on fibronectin, poly-D-lysine, collagen or laminin coated coverglasses and non coated coverglass (Ctrl) were analysed by immunoblot for p110δ expression using p110δ-specific antibody (sc7176). Actin was used as a loading control. Relative densitometry analysis of p110δ from three different experiments was analysed and presented in histograms below. Values are expressed as mean±s.e.m. (f) Total RNA from cells inewere analysed by qRT–PCR for p110δ expression and normalized to GAPDH. Values from three independent experiments are expressed as mean±s.e.m. *P<0.05, **P<0.001 (Student’st-test). (g) Total RNA from cells grown or not on Matrigel for 4 days were analysed by qRT–PCR for p110δ expression and normalized to GAPDH (see Methods). Values from three independent experiments are expressed as mean±s.e.m. *P<0.05 (Student’st-test). Figure 6: ECM regulates p110δ expression. ( a ) MDCK cells transfected or not with 1 μg of Myc 2-p110δ were grown on matrigel and fixed after 24 h for AMIS, after 48 h for PAP and after 72 h for open lumen. Cells were stained with laminin (green), actin (red) and Hoechst (blue) as indicated in the pictures. A confocal section through the middle of cyst is shown. Scale bar, 10 μm. 3D reconstruction from all xz sections is presented in a grey background. Laminin signal intensity of individual cell is analysed with ImageJ software for 30 cells and represented as histogram in b . Values are expressed as mean±s.e.m. *** P <0.0001 (Student’s t -test). ( c , d ) Same as a and b , respectively, for type IV collagen staining (green) and signal intensity. ( e ) MDCK cells grown for 24 h on fibronectin, poly- D -lysine, collagen or laminin coated coverglasses and non coated coverglass (Ctrl) were analysed by immunoblot for p110δ expression using p110δ-specific antibody (sc7176). Actin was used as a loading control. Relative densitometry analysis of p110δ from three different experiments was analysed and presented in histograms below. Values are expressed as mean±s.e.m. ( f ) Total RNA from cells in e were analysed by qRT–PCR for p110δ expression and normalized to GAPDH. Values from three independent experiments are expressed as mean±s.e.m. * P <0.05, ** P <0.001 (Student’s t -test). ( g ) Total RNA from cells grown or not on Matrigel for 4 days were analysed by qRT–PCR for p110δ expression and normalized to GAPDH (see Methods). Values from three independent experiments are expressed as mean±s.e.m. * P <0.05 (Student’s t -test). Full size image Next we examined the possible role of ECM in regulating the expression of p110δ. To this end, multiwell plates were either coated or not with various ECM components, including: type I collagen, laminin, fibronectin or poly- D -Lysine. MDCK cells were plated for 24 h on the different ECM-coated supports and analysis for the impact of different ECM components on p110δ expression was performed by immunoblotting. P110δ expression is increased in response to cell interactions with all ECM substrates analysed in comparison with expression levels of p110δ expression detected on an untreated support (Ctrl; Fig. 6e ). Similar data were obtained using RT–PCR analysis of p110δ gene expression under these treatments ( Fig. 6f ). Moreover, we demonstrated that p110δ mRNA level increased significantly in cells grown on matrigel ( Fig. 6g ). Although there were no statistically significant differences between the effects of the different ECM proteins tested in our experimental conditions at the p110δ protein level, collectively these data are supportive of a role for ECM components in positively regulating p110δ expression. Depletion of p110δ inverts polarity and impairs BM assembly To validate the specificity of the observed effects with the pharmacological inhibitors of p110δ, we used three different short interfering RNAs (siRNAs; si1, si2 and si3) that isoform specifically reduced the abundance of the p110δ transcript, since there was no effect of these siRNAs on the mRNA levels of p110α, β and γ ( Fig. 7a ). The mechanism by which PtdIns(3,4,5)P 3 regulates cellular signalling was first revealed for Akt [38] . Thus, we analysed the effects of p110δ expression on the phosphorylation status of Akt. No significant change in pAkt was observed after the depletion of p110δ using each of the three different siRNAs and on the stimulation of cells with epidermal growth factor ( Supplementary Fig. 6 ). Consistent results were obtained on the overexpression of Myc-tagged p110δ, strongly suggesting that p110δ is not a key signalling molecule for Akt phosphorylation ( Supplementary Fig. 6 ). Similar data were previously observed in endothelial cells [39] . 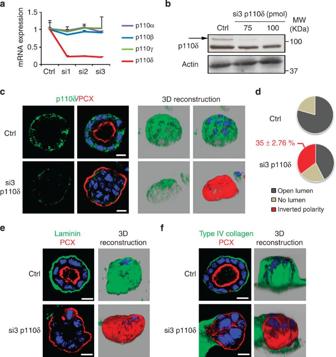Figure 7: p110δ knockdown alters laminin and type IV collagen assembly and leads to inverted polarized cyst formation. (a) MDCK cells were transfected with 100 pmol of three different p110δ-specific siRNA (si1, si2 and si3) for 48 h. Total RNA was analysed by qRT–PCR for p110δ, p110α, p110β and p110γ and normalized to GAPDH (see Methods). Control (Ctrl) corresponds to cells treated with transfection reagents only. Values are expressed as mean±s.e.m. of four triplicate independent experiments. (b) Immunoblot analysis of p110δ using p110δ-specific antibody (sc7176), in MDCK cells transfected or not with 75 and 100 pmol of p110δ siRNA. Actin was used as a loading control. (c) MDCK transfected as inawith si3 or ctrl cells were grown in Matrigel for 96 h to form cysts and then stained for p110δ (green) using p110δ-specific antibody (ab32401), PCX (red) and Hoechst (blue). Single confocal section through the middle of the cyst is shown. Scale bar, 10 μm. 3D reconstruction from allxzsections is presented in the right column in grey background. (d) Quantification of open lumen, no lumen and inverted polarized cysts from three independent experiments was presented in pie. The percentage±s.e.m. of inverted polarized cyst is indicated above the pie. (e) MDCK cysts incwere stained for laminin (green), PCX (red) and Hoechst (blue). A confocal section through the middle of cyst is shown. Scale bar, 10 μm. 3D reconstruction from allxzsections is presented in the right column in grey background. (f) MDCK cells incwere stained for type IV collagen (green), PCX (red) and Hoechst (blue). A confocal section through the middle of cyst is shown. Scale bar, 10 μm. 3D reconstruction from allxzsections is presented in the right column in grey background. Figure 7: p110δ knockdown alters laminin and type IV collagen assembly and leads to inverted polarized cyst formation. ( a ) MDCK cells were transfected with 100 pmol of three different p110δ-specific siRNA (si1, si2 and si3) for 48 h. Total RNA was analysed by qRT–PCR for p110δ, p110α, p110β and p110γ and normalized to GAPDH (see Methods). Control (Ctrl) corresponds to cells treated with transfection reagents only. Values are expressed as mean±s.e.m. of four triplicate independent experiments. ( b ) Immunoblot analysis of p110δ using p110δ-specific antibody (sc7176), in MDCK cells transfected or not with 75 and 100 pmol of p110δ siRNA. Actin was used as a loading control. ( c ) MDCK transfected as in a with si3 or ctrl cells were grown in Matrigel for 96 h to form cysts and then stained for p110δ (green) using p110δ-specific antibody (ab32401), PCX (red) and Hoechst (blue). Single confocal section through the middle of the cyst is shown. Scale bar, 10 μm. 3D reconstruction from all xz sections is presented in the right column in grey background. ( d ) Quantification of open lumen, no lumen and inverted polarized cysts from three independent experiments was presented in pie. The percentage±s.e.m. of inverted polarized cyst is indicated above the pie. ( e ) MDCK cysts in c were stained for laminin (green), PCX (red) and Hoechst (blue). A confocal section through the middle of cyst is shown. Scale bar, 10 μm. 3D reconstruction from all xz sections is presented in the right column in grey background. ( f ) MDCK cells in c were stained for type IV collagen (green), PCX (red) and Hoechst (blue). A confocal section through the middle of cyst is shown. Scale bar, 10 μm. 3D reconstruction from all xz sections is presented in the right column in grey background. Full size image Next MDCK cells treated or not with siRNA (si3) were grown on matrigel to form cysts. The specificity of si3 was further verified by immunoblot ( Fig. 7b ). In control cysts, p110δ was found at the basal membrane (as described in Fig. 3 ) and the signal was profoundly reduced in cysts from siRNA-treated cells confirming a specific signal for the antibody ( Fig. 7c ). Consistent with our inhibitors studies, PCX was located at the cyst periphery in siRNA-treated cysts as evidenced by the 3D reconstruction of the confocal data ( Fig. 7c right panels). The tight junctions marker (ZO-1), normally present at the tip of β-catenin positive cell–cell contacts in control cysts was now found at the basal region of cysts formed from siRNA-treated cells ( Supplementary Fig. 7 ). Analysis of confocal data indicated that 35% (±2.76%) of the total cysts presented an inversion of polarity, with PCX present at the external surface ( Fig. 7d ). These data are consistent with those obtained on treatment of cells with IC87114 or CAL-101 ( Supplementary Fig. 1 ). The percentage of cysts with inverted polarity observed in our study is also consistent with the outcomes (30–50%) recently published in different studies [34] , [40] . Moreover, in the p110δ depleted and inverted polarized cysts, no laminin ( Fig. 7e ), or type IV collagen ( Fig. 7f ), was detected at the cyst periphery. Taken together, these data confirmed that p110δ is required for the orientation of the apico-basal axis, lumen formation, laminin and type IV Collagen assembly through an inside-out signal. p110δ is required for focal adhesion stability The spatial cues from cell adhesion to the ECM are mediated primarily through integrins, an adhesion molecule superfamily of heterodimeric transmembrane proteins composed of α and β subunits with variable affinities towards the different ECM proteins and specific roles in ECM assembly and remodelling [41] , [42] . β1 integrins are widely expressed in epithelial cells, and studies using both function-blocking antibodies and genetic deletion approaches have revealed that they control BM deposition, control BM assembly and have a central role in establishing apico-basal polarity [33] , [43] . The β1 integrin is involved in different combinations with many alpha subunits including α 2 and α 5 showing a preference for collagen and fibronectin receptors, respectively. The α2β1 integrin combinations are also able to interact with laminin [41] . Therefore, we analysed the β1, α 2 and α 5 integrins in p110δ-disrupted cells. In control cysts, the staining of β1 integrin, α 2 integrin and α 5 integrin were mainly detected at the basolateral membrane of polarized cysts. Knockdown of p110δ expression using siRNA as well as treatment of cells using CAL-101 dramatically reduced the staining for the different integrins and particularly of β1 integrin, where the signal was largely abolished ( Supplementary Fig. 8 ). The binding of integrins to ligand initiates the connection between the cytoskeleton and the ECM and contributes to the recruitment of additional cytoskeletal and signalling proteins such as talin, vinculin and paxillin that create focal adhesions and regulate cell shape and polarity [1] , [44] . Thus, to further characterize the effect of p110δ on ECM signalling and focal adhesions, we examined both paxillin and vinculin expression and organization. In control cysts, paxillin was organized at the basolateral membrane adjacent to laminin, while the protein became more cytoplasmic and diffuse on treatment of cysts with IC87114 ( Fig. 8a,b ). Similar observations were made for vinculin ( Fig. 8c,d ), indicating that p110δ activity regulates paxillin and vinculin subcellular localization and partly co-localized with them ( Supplementary Fig. 9 ). 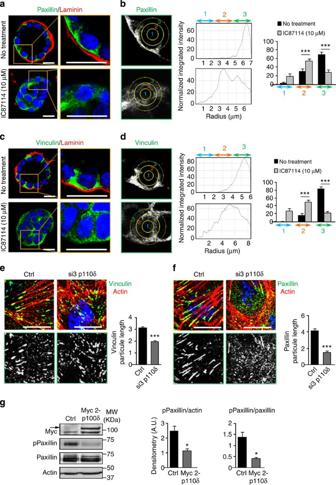Figure 8: p110δ regulates the membrane localization of paxillin and vinculin and focal adhesion organization. (a,c) MDCK cells treated or not with 10 μM of IC87114 were grown on Matrigel for 96 h to form cysts, and stained for paxillin (a) and vinculin (c) (green), laminin (red) and Hoechst (blue). A confocal section through the middle of cyst is shown. Scale bar, 10 μm. A higher magnification of the data is presented in the right column. (b,d) The distribution of paxillin (b) and vinculin (d) signal was analysed by ImageJ software in an individual cell from a cyst as inFig. 4b. The total intensity in each band was calculated from 20 cells was represented as histogram. Values are expressed as mean±s.e.m. ***P<0.0001 (Student’st-test). (e) MDCK cells transfected with 100 pmol of p110δ-specific siRNA (si3) or control (Ctrl) cells were grown for 48 h on coverglasses and stained for vinculin (green), actin (red) and Hoechst (blue) as indicated on the figures. Scale bar, 10 μm. Vinculin staining alone is presented in black and white in the bottom panels. Vinculin particle length is measured with ImageJ for 30 cells from three independent experiments and presented in histogram on the right part of the figure. Values are expressed as mean±s.e.m. and ***P<0.0001 (Student’st-test). (f) Same as ine, for paxillin staining and analysis. (g) Paxillin and phosphorylated paxillin (pPaxillin) were analysed by immunoblot on lysates from cells transfected or not with 1 μg of Myc2-p110δ. Actin was used as loading control. Densitometry analysis of the ratio of pPaxillin to actin and pPaxillin to total Paxillin from three different experiments was analyzed and presented in histograms. Values are expressed as mean±s.e.m. and *P<0.05 (Student’st-test). Figure 8: p110δ regulates the membrane localization of paxillin and vinculin and focal adhesion organization. ( a , c ) MDCK cells treated or not with 10 μM of IC87114 were grown on Matrigel for 96 h to form cysts, and stained for paxillin ( a ) and vinculin ( c ) (green), laminin (red) and Hoechst (blue). A confocal section through the middle of cyst is shown. Scale bar, 10 μm. A higher magnification of the data is presented in the right column. ( b , d ) The distribution of paxillin ( b ) and vinculin ( d ) signal was analysed by ImageJ software in an individual cell from a cyst as in Fig. 4b . The total intensity in each band was calculated from 20 cells was represented as histogram. Values are expressed as mean±s.e.m. *** P <0.0001 (Student’s t -test). ( e ) MDCK cells transfected with 100 pmol of p110δ-specific siRNA (si3) or control (Ctrl) cells were grown for 48 h on coverglasses and stained for vinculin (green), actin (red) and Hoechst (blue) as indicated on the figures. Scale bar, 10 μm. Vinculin staining alone is presented in black and white in the bottom panels. Vinculin particle length is measured with ImageJ for 30 cells from three independent experiments and presented in histogram on the right part of the figure. Values are expressed as mean±s.e.m. and *** P <0.0001 (Student’s t -test). ( f ) Same as in e , for paxillin staining and analysis. ( g ) Paxillin and phosphorylated paxillin (pPaxillin) were analysed by immunoblot on lysates from cells transfected or not with 1 μg of Myc2-p110δ. Actin was used as loading control. Densitometry analysis of the ratio of pPaxillin to actin and pPaxillin to total Paxillin from three different experiments was analyzed and presented in histograms. Values are expressed as mean±s.e.m. and * P <0.05 (Student’s t -test). Full size image We next investigated focal adhesions by growing cells on glass to better visualize these structures. Under such conditions, vinculin localized at the ends of actin stress fibres, whereas in cells treated with p110δ siRNA vinculin formed smaller and punctuate foci dispersed in the cytoplasm ( Fig. 8e ). A prominent effect of p110δ siRNA was also observed on paxillin distribution ( Fig. 8f ). The level of tyrosine phosphorylation of paxillin is known to positively correlate to dynamism of adhesion sites [45] . Decreased paxillin phosphorylation reduces the turnover of focal contacts and their stabilization, which is required for cell differentiation and polarization. Immunoblotting revealed a decrease in the phosphorylation of paxillin on tyrosine-118 (pPaxillin) on p110δ overexpression ( Fig. 8g ), suggesting that p110δ could promote the stabilization of focal contacts at the basal membrane. p110δ co-localizes with β-DG and regulates its localization Although the most intensively studied receptors for ECM compounds are integrins, dystroglycan (DG) is another high-affinity laminin receptor, originally identified in studies on muscular dystrophy [46] , [47] . DG is a heterodimeric glycoprotein that consists of a transmembrane β-subunit and a non-covalently associated, extracellular α-subunit. The cytoplasmic domain is linked to the actin cytoskeleton, whereas the extracellular domain is implicated in laminin assembly and subsequently shown to play important roles in the cell–ECM interactions, BM assembly, cell polarity and morphogenesis [48] , [49] , [50] , [51] . Consistent with the absence of ECM at the periphery of inverted polarized cysts, we hypothesized that DG could also be regulated by p110δ. In control cysts, β-dystroglycan (β-DG) was clearly visible at the basal membrane at the ECM contacts and some co-localization with p110δ was observed, which increased on p110δ overexpression ( Fig. 9a ). In contrast, siRNA-mediated p110δ knockdown strongly reduced β-DG membrane localization with a drastic reduction of the co-localization signal ( Fig. 9a ). Treatment of cysts with IC87114 yielded similar results to those observed using the isoform specific siRNA strategy ( Fig. 9b ). We further reinforced these observations by using CAL-101 to inhibit p110δ enzymatic activity. As shown in 2D and 3D reconstructions, the β-DG signal that outlined cell periphery in untreated cysts disappeared and instead accumulated at the bottom of the cysts ( Fig. 9c ). Collectively, these data emphasize the functional contribution of p110δ in β-DG localization at the basolateral membrane. Next we investigated the existence of a feedback control loop of β-DG on p110δ expression and localization. In concert with our predictions, siRNA-mediated knockdown of β-DG led to cysts exhibiting inversion of polarity and to the absence of laminin accumulation at the cyst periphery ( Fig. 9d,e ). Under these experimental conditions, p110δ was found mostly in the cytoplasm ( Fig. 9f ). In conclusion, these data demonstrate that p110δ localization at the basal membrane is also regulated by an outside-in signal from the ECM via β-DG that drives the orientation of polarity axis. 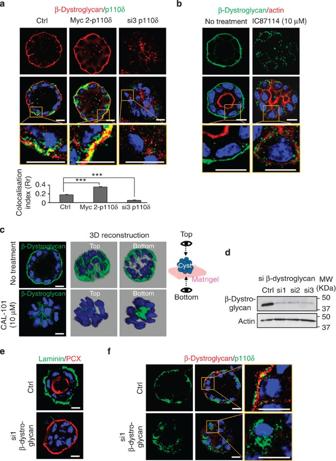Figure 9: p110δ is required for the membrane localization of β-dystroglycan (β-DG). (a) MDCK cells transfected with 1 μg of Myc 2-p110δ cDNA or 100 pmol of si3 were grown to form cysts, stained for β-DG (red), p110δ (green) using p110δ-specific antibody (ab32401) and Hoechst (blue) as indicated on the figures. Confocal section through the middle of a cyst is shown for β-DG (red) and the merged picture with p110δ. A higher magnification of the merged picture is represented in the bottom rows. Scale bar, 10 μm. Data (mean±s.e.m.) for measure of co-localization calculated from 15 cysts using ImageJ software as described in Methods section were indicated in histogram below the panels. (b) MDCK cysts, treated or not with 10 μM of IC87114 for 72 h were stained for β-DG (green), actin (red) and Hoechst (blue) as indicated in the pictures. Confocal section through the middle of cyst is shown. A higher magnification is represented in the bottom row. Scale bar, 10 μm. (c) MDCK cells, treated or not with 10 μM of CAL-101 for 72 h were grown on Matrigel to form cyst and stained for β-DG (green) and Hoechst (blue). Confocal section through the middle of cyst is shown, and 3D reconstruction from allxzsections is presented in grey background. Two sides of view (top and bottom) were shown as illustrated at right. (d) Immunoblot of β-DG in MDCK cells transfected with 100 pmol of three different β-DG specific siRNA (si1, si2 and si3) and control cells (Ctrl). Actin served as a loading control. (e) MDCK cells transfected for 24 h with si1 β-DG as indwere grown in Matrigel for 96 h to form cysts and then stained for laminin (green), PCX (red) and Hoechst (blue). Single confocal section through the middle of cyst is shown. (f) MDCK cysts inewere stained for β-DG (red), p110δ (green) using p110δ-specific antibody (ab32401) and Hoechst (blue). Single confocal section through the middle of cyst is shown. A higher magnification is presented in the right panels. Scale bar, 10 μm. Figure 9: p110δ is required for the membrane localization of β-dystroglycan (β-DG). ( a ) MDCK cells transfected with 1 μg of Myc 2-p110δ cDNA or 100 pmol of si3 were grown to form cysts, stained for β-DG (red), p110δ (green) using p110δ-specific antibody (ab32401) and Hoechst (blue) as indicated on the figures. Confocal section through the middle of a cyst is shown for β-DG (red) and the merged picture with p110δ. A higher magnification of the merged picture is represented in the bottom rows. Scale bar, 10 μm. Data (mean±s.e.m.) for measure of co-localization calculated from 15 cysts using ImageJ software as described in Methods section were indicated in histogram below the panels. ( b ) MDCK cysts, treated or not with 10 μM of IC87114 for 72 h were stained for β-DG (green), actin (red) and Hoechst (blue) as indicated in the pictures. Confocal section through the middle of cyst is shown. A higher magnification is represented in the bottom row. Scale bar, 10 μm. ( c ) MDCK cells, treated or not with 10 μM of CAL-101 for 72 h were grown on Matrigel to form cyst and stained for β-DG (green) and Hoechst (blue). Confocal section through the middle of cyst is shown, and 3D reconstruction from all xz sections is presented in grey background. Two sides of view (top and bottom) were shown as illustrated at right. ( d ) Immunoblot of β-DG in MDCK cells transfected with 100 pmol of three different β-DG specific siRNA (si1, si2 and si3) and control cells (Ctrl). Actin served as a loading control. ( e ) MDCK cells transfected for 24 h with si1 β-DG as in d were grown in Matrigel for 96 h to form cysts and then stained for laminin (green), PCX (red) and Hoechst (blue). Single confocal section through the middle of cyst is shown. ( f ) MDCK cysts in e were stained for β-DG (red), p110δ (green) using p110δ-specific antibody (ab32401) and Hoechst (blue). Single confocal section through the middle of cyst is shown. A higher magnification is presented in the right panels. Scale bar, 10 μm. Full size image PI3Ks transmit signals from transmembrane receptors such as receptor tyrosine kinases and G-protein-coupled receptors to control a diverse array of signalling pathways through spatiotemporal recruitment of multiple effectors containing PI-specific binding domains. Thus, they regulate key cellular processes including, cell migration, proliferation, differentiation and survival and as such are targeted for intensive research across the fields of inflammation, immunity, cancer and metabolic diseases [12] , [38] , [52] . PtdIns(3,4,5)P 3 , the major product of class I PI3K, plays a crucial role in the generation of epithelial polarity [16] . In line with these previous publications, our results indicate that all of the isoforms of class IA PI3Ks participate in MDCK cyst morphogenesis and the development of epithelial polarity ( Fig. 1 ). The different phenotypes observed using specific isoform inhibitors ( Fig. 1 ) suggested that each of the isoforms has a particular function at a different step of the intricate polarity programme. Unexpectedly, only inhibition of the isoform delta, the least abundantly expressed isoform in MDCK cells, affects the initiation of lumen formation and orientation of the apico-basal polarity axis. Through the use of mice with inactivated p110δ and also selective inhibitors, such as the IC87114 and CAL-101 compounds, the p110δ isoform of PI3K has been extensively studied in leukocytes and is designated as a potential therapeutic target in immunity, inflammation and haematological malignancies [53] , [54] , [55] , [56] , [57] . Nevertheless, mice lacking PI3Kδ have thus far only been studied under basal conditions. Yet, mice lacking PI3Kδ have thickened intestinal mucosa with hyperplasic glands and mixed inflammatory infiltration of the lamina propria [54] . Even though these effects were attributed to the neutrophilic inflammation, one could not exclude an effect on the epithelial cells, which composed the mucosa. Thus, further in vivo studies were required to determine the polarity defects associated with PI3Kδ knockdown in vivo . The preponderance of studies of p110δ function in haematological systems has contributed to the dogma of a restricted role of p110δ in cells of haematopoietic lineage. Of interest, the development of PI3K isoform-selective inhibitors [12] , [58] , [59] , [60] , [61] and the determination of its crystal structure [62] has advanced the emerging studies of p110δ function in non-haematopoietic cells. Still, most of these studies are related to p110δ expression in cancer where p110δ has been shown to be the predominant isoform expressed in different human solid tumour cells including; glioblastoma, neuroblastoma, prostate carcinoma and breast cancer [63] . A recent report indicated a somatic mutation in PI3Kδ that is associated with recurrent infections and airway damage [64] . Thus, a better understanding of the regulation and function of p110δ in non-haematopoietic cells and their connections to oncogenesis is both warranted and timely. In the present study, we provided important insights into the fundamental role of p110δ in the establishment of apico-basal polarity axis and lumen formation in MDCK cells. It is generally accepted that the acquisition of epithelial polarity depends on signalling generated through cell interactions with neighbouring cells and with the surrounding ECM [4] , [5] , [31] . Integrins are critical components of this signalling pathway and are known modulators of PI3K and PtdIns(3,4,5)P 3 levels [33] , [65] , [66] . Integrin-mediated PI3K activation induces Rac1 activation and thereby organizes the actin cytoskeleton and recruitment of adaptor proteins within adhesion complexes (that contain a large set of proteins, including paxillin and vinculin [67] ). Our data revealed a role for p110δ in the establishment of the apico-basal polarity axis acting via outside-in signalling cascade that is triggered by cell adhesion to the ECM where it acts to establish apico-basal polarity axis and lumen formation that are crucial to epithelial morphogenesis. Of note, previous studies have reported the contribution of other isoforms of PI3K, including p110α and p110β, in the control of integrin signalling [66] , [68] and Rho GTPases [69] . Thus, the contributions of the other PI3K isoforms in epithelial organization were not excluded. We also demonstrated that the inhibition of p110δ activity or knockdown of its expression affected laminin and type IV collagen assembly at the cyst periphery. Moreover, these treatments profoundly reduced the integrin expression and impaired both paxillin and vinculin focal distribution, where instead these proteins were found diffuse in the cytoplasm ( Fig. 8 ). Furthermore, we showed that different ECM proteins positively regulated p110δ expression ( Fig. 6e,f ). Together these data also demonstrated a role for p110δ in inside-out signalling to control basal membrane organization. However, further investigations are necessary to establish the precise influence of the type of ECM component, the concentration and the stiffness of the ECM on p110δ expression and on the cell polarization process in general. Using a specific antibody, we demonstrated the presence of PtdIns(3,4,5)P 3 at the basolateral membrane of polarized cysts as previously reported [21] . Interestingly, the treatment of cysts with IC87114 strongly reduced PtdIns(3,4,5)P 3 accumulation at the membrane. It is noteworthy that the intensity of the staining for PtdIns(3,4,5)P 3 in the inhibitor-treated cells was not impacted, which indicates that p110δ is not the only enzyme responsible for PtdIns(3,4,5)P 3 production in our system. However, the displacement of PtdIns(3,4,5)P 3 from the basal membrane on treatment with IC87114 suggested that p110δ is the PI3K isoform activated at the site of ECM contact during initiation of the epithelial cell polarization process. These findings are in concordance with our previous description of PtdIns(3,4,5)P 3 as a compass for cell polarization and as a regulator of basolateral membrane formation [21] . PI3K is a known effector of small family of GTPases including Rac1 and the contribution of PI3K downstream of the laminin signal in the regulation of cell polarity has been reported [36] . However, it must be noted that the majority of the previous studies were performed using the broad-spectrum inhibitors of class I PI3K, including LY294002 or wortmannin, and as such they do not enable the identification of the specific PI3K isoform involved. Here we provide the first evidence that the p110δ isoform of PI3K regulates Rac1 activation in the context of apico-basal polarization in epithelia ( Supplementary Fig. 5 ). DG is another receptor for laminin that plays critical roles in BM organization and epithelial polarity through the assembly of extracellular laminin [47] , [48] , [51] . However, the underlying mechanisms remain poorly understood. This study revealed that p110δ regulated the maintenance of β-DG at the basal membrane and reciprocally β-DG controlled membrane localization of both p110δ and its lipid product PtdIns(3,4,5)P 3 . DG regulates actin organization and participates in Rac1 activation [70] , suggesting that p110δ could act at the crossroads between integrin and DG mediated ECM signalling to drive the cytoskeleton organization and Rac1 activation that are required for spatial orientation of polarity. However, Rac1 does not seem to be the only downstream effector of ECM/integrin signalling during cell polarization [40] . Understanding the source of this apparent discordance regarding the role of Rac1 requires further investigation. There are important changes in ECM composition according to the cell type and the differentiation stage [70] . Moreover, there are different receptors for the myriad ECM proteins and almost 100 different proteins are present in focal complexes, including signalling molecules and adaptors. The apparent complexity of cell–matrix adhesions suggests that only a subset of proteins participate in different signalling pathways, clearly indicating that more studies are required to elucidate the intricacies of the signalling pathways that link cell/ECM contacts to the polarization process. PAR-1, a downstream target of the aPKC-PAR-3-PAR-6 complex, regulates the basolateral localization of the DG complex [49] . At the early stage of cyst formation, PCX is localized at the cell periphery in contact with the ECM. It was shown that membrane trafficking regulated by Rab proteins in cooperation with Par3–aPKC drives vesicles to the apical surface to initiate lumen formation [27] . We have shown here that inhibition of p110δ activity induced maintenance of PCX at the cell periphery ( Figs 1 and 3 ). Thus, one could speculate that PI3Kδ signalling could play an important role in the targeting of these apical cargoes through determination of the polarity axis, although this remains to be determined. In epithelial cells, dynamic remodelling of the ECM is essential for the development and normal tissue homeostasis. However, loss of polarity and uncontrolled ECM remodelling often leads to fibrotic diseases and cancer. Thus, the analysis of p110δ in carcinoma, in particular those associated with fibrosis, will be of potential interest for cancer research. Inhibitors TGX115, AS-605240, PI-103 and IC87114 (Symansis) were from Kevan Shokat (University of California San Francisco, US) and CAL-101 was purchased from Selleck Chemicals. Stock solutions of the different inhibitors were prepared in dimethyl sulfoxide and the used concentrations were mentioned in the figure legends. Antibodies Two primary antibodies were used for p110δ, the rabbit anti p110δ from Santa Cruz sc7176 (1:500 dilution is used for immunoblot and 1:50 dilution is used for immunofluorescence staining in Supplementary Fig. 3 ) and the anti-PI 3-Kinase p110δ antibody from Abcam ab32401 (1:50 dilution is used for immunofluorescence only). The other antibodies used were: Mouse anti PtdIns(3,4,5)P 3 (Echelon Biosciences (Tebu-Bio Z-G345), 1:50), mouse Anti β-distroglycan (Abcam ab49515, 1:50 for immunofluorescence and 1:1,000 for immunoblot), rabbit anti type IV collagen (Abcam ab6586, 1:100 for immunofluorescence), Rabbit anti β-catenin (Santa Cruz sc-7199, 1:100 for immunofluorescence), mouse anti integrin β1 (Santa Cruz sc-18887, 1:50 for immunofluorescence), mouse anti paxillin (Cell Signaling 612642, 1:100 for immunofluorescence and 1:1,000 for immunoblot), rabbit anti phospho paxillin Tyr118 (Cell Signaling 2541, 1:100 for immunofluorescence and 1:1,000 for immunoblot), rabbit anti Laminin (Sigma L9393, 1:100), mouse anti Vinculin (Sigma 031M4818, 1:100), goat anti Actin (I-19) (Santa Cruz sc-1616, 1:2,000), mouse Anti Myc (Sigma M4439 1:100 for immunofluorescence and 1:1,000 for immunoblot), mouse anti integrin α2 (BD biosciences V75320, 1:50) and mouse anti integrin α5 (BD biosciences I55220, 1:50). The mouse anti PCX antibody (1:1,000) was from George Ojakian (University of New York Downstate Medical Center), USA. Rat anti ZO-1 antibody (dilution 1:100) was from Bruce Stevenson (University of Alberta, Edmonton, AB, Canada). Secondary antibodies used were highly cross-absorbed anti-mouse, anti-rabbit or anti-goat Alexa Fluor 546 and 488 (Invitrogen, 1:100). Actin was stained with Alexa Fluor 546 phalloidin (Invitrogen A22283, 1:100) and nuclei with Hoechst 34580 (Invitrogen H21486, 1:5,000). Secondary horseradish peroxidase antibodies were anti-goat, anti-rabbit or anti-mouse (Sigma, 1:2,000). Cells and 3D culture MDCK (Madin–Darby Canine Kidney) cells (Keith Mostov, UCSF, San Francisco), were cultured in minimal essential medium containing Earle’s balanced salt solution supplemented with 5% fetal bovine serum and 1% of penicillin/streptomycin solution (10,000 U ml −1 /10,000 μg ml −1 ) at 37 °C in 5% CO2, 95% air. For 3D culture, MDCK cells were trypsinized as 15,000 single cells ml −1 in 2% Matrigel (BD), 500 μl of cells were plated in each well of eight-well Lab-Tek II chamber slides (Thermo Fisher Scientific) precovered with Matrigel and grown for 4 days until cysts with lumen formed. The human HeLa cells (from ATCC) were cultured in Dulbecco’s modified Eagle’s Medium containing 4.5 g l −1 glucose supplemented with 10% heat-inactivated fetal bovine serum, 1% nonessential amino acids and 1% penicillin/streptomycin. To analyze the effect of the ECM on p110δ, MDCK cells were plated for 24 h on 8-well CultureSlides precovered with Fibronectin, poly- D -Lysine, type I Collagen or Laminin (from BD Biosciences). SiRNA, plasmids and cell transfection The specific p110δ duplex RNAi used were: si1:5′-CAACAUCCAGCUAAACAAA[dT][dT]-3′ and 5′-UUUGUUUAGCUGGAUGUUG[dT][dT]-3′, si2: 5′-GAAUAACAGUGAGAAAUUU[dT][dT]-3′ and 5′-AAAUUUCUCACUGUUAUUC[dT][dT]-3′, si3: 5′-CACUUUAUGCUGUGAUCGA[dT][dT]-3′ and 5′-UCGAUCACAGCAUAAAGUG[dT][dT]-3′. The specific β-DG duplex RNAi used were: si1: 5′-CCUUCUAUGACCACGAGGA[dT][dT]-3′ and 5′-UCCUCGUGGUCAUAGAAGG[dT][dT]-3′, si2: 5′-GGCAUAUUGCCAACAAGAA[dT][dT]-3′ and 5′-UUCUUGUUGGCAAUAUGCC[dT][dT]-3′, si3: 5′-GUUUAUCUGCACACAGUCA[dT][dT]-3′ and 5′-UGACUGUGUGUGCAGAUAAAC[dT][dT]-3′. Human p110δ cDNAs were from Bart Vanhaesebroeck, University College London, UK (MTA-1004.0-0-Acad-OUT-NB-4214), either pMT-SM-human p110δ-WT-3Myc (Myc 1-p110δ), pCDNA3tk-human p110δ-WT-3Myc (Myc 2-p110δ) or the untagged pMT-SM-human p110δ (UT-p110δ). For transfection, MDCK cells seeded at low density (1 × 10 4 cells cm −2 ) were transfected with 100 pmol of specific siRNA or 1 μg cDNA using jetPRIME (Ozyme) according to the manufacturer’s instructions. For 3D culture, 24 h after transfection, cells were detached with trypsin and plated on Matrigel for 4 days as indicated above. Immunofluorescent staining MDCK cells were rinsed with ice cold Dulbecco’s PBS (DPBS) and fixed with 3.7% paraformaldehyde for 30 min. Samples were permeabilized and saturated with DPBS supplemented with 0.7% fish gelatin and 0.025% saponin for 30 min at 37 °C and then incubated with primary antibodies. After the washes, staining was performed with secondary fluorescent antibodies, phalloidin and Hoechst. Samples were observed with a Leica TCS SP5 AOBS tandem 30 confocal microscope. Images were collected as TIF files and analysed with PhotoShop. Immunoblot Cells were lysed in 1 × lysis buffer (20 mM Tris–HCl (pH 7.5), 100 mM NaCl, 1 mM EDTA, and 1% Triton-X-100) containing 1 × complete protease and phosphatase inhibitor cocktail (Roche diagnostics). An aliquot of quantitated proteins was resolved on SDS-polyacrylamide gel electrophoresis and then electrotransferred onto polyvinylidene difluoride membrane. After transfer, the membrane was saturated in DPBS containing 0.1% Tween 20 and 5% milk. Primary antibodies were added overnight at 4 °C. After washes in the presence of DPBS, appropriate secondary antibodies coupled with peroxidase were added. Immunoblotting was revealed with chemiluminescent peroxidase substrate (Chemiluminescent Peroxidase Substrate-3, Sigma-Aldrich) and exposure on Kodak Biomax Light film or with Gbox. Blot scans are presented cropped in figures and at least one marker position is presented. Uncropped scans are supplied in Supplementary Fig. 10 . Rac1 activation assay Rac1 activation was quantified using G-LIZA Biochem Kit (luminescence based) from TEBU-BIO as described by the manufacturer. In brief, cells lysates as described above for immunoblot (1 μg μl −1 for protein concentration) were incubated in the affinity wells for 30 min at 40 °C. Antigen-presenting buffer was added for 2 min. Primary and secondary antibodies were incubated for 45 min at room temperature. Intensity was measured by luminometer at 0.3 s with horseradish peroxidase detection reagent. Cell lyses buffer was used as blank control (RLU, relative light unit). Quantitative reverse transcription–PCR Total RNA was isolated using RNeasy Mini Kit 50 (Qiagen) and applied to reverse transcription using RevertAid First Strand cDNA Synthesis Kit (Fermentas). The cDNA was analysed by qPCR using Quanti Tect SYBR Green PCR Kit (QIAGEN) with 7500 Fast Real-Time PCR System (Applied Biosystems). Reaction parameters were 50 °C for 30 min, 95 °C for 15 min, followed by 45 cycles of 94 °C for 15 s, 55 °C for 30 s and 72 °C for 30 s. The triplicate mean values were calculated using GAPDH gene transcription as reference for normalization. The primers used are indicated in Supplementary Table 1 . Image analysis Images obtained by confocal microscopy were analysed by Icy software for 3D reconstruction. For co-localization analysis, images were treated by ImageJ software, the plugin ‘Intensity Correlation Analysis’ was used. Co-localization index was obtained via Pearson’s correlation coefficient ( Rr ). The values for Pearson’s coefficient range from 1 to −1. A value of 1 represents perfect correlation, −1 represents perfect exclusion and zero represents random localization. For intensity distribution in cells, the plugin ‘Radial profil’ was used. For analysis of a cyst, a circle was defined at the periphery of each cell and the plugin produces a profile plot of normalized integrated intensities around concentric circles as a function of distance from a point in the image, considered here as the centre of the cell. The concentric circles were assembled in three circle bands with equal radius. The intensity in each band was calculated from the total integrated intensities around concentric circles present in the band. Statistical analyses All values are expressed as mean±s.e.m. Comparison of mean values was conducted with unpaired Student’s t -test. Statistical significance was determined at * P <0.05, ** P <0.001 and *** P <0.0001. How to cite this article: Peng, J. et al. Phosphoinositide 3-kinase p110δ promotes lumen formation through the enhancement of apico-basal polarity and basal membrane organization. Nat. Commun. 6:5937 doi: 10.1038/ncomms6937 (2015).